Anthropogenic radionuclides in atmospheric air over Switzerland during the last few decades The atmospheric nuclear testing in the 1950s and early 1960s and the burn-up of the SNAP-9A satellite led to large injections of radionuclides into the stratosphere. It is generally accepted that current levels of plutonium and caesium radionuclides in the stratosphere are negligible. Here we show that those radionuclides are present in the stratosphere at higher levels than in the troposphere. The lower content in the troposphere reveals that dry and wet deposition efficiently removes radionuclides within a period of a few weeks to months. Since the stratosphere is thermally stratified and separated from the troposphere by the tropopause, radioactive aerosols remain longer. We estimate a mean residence time for plutonium and caesium radionuclides in the stratosphere of 2.5–5 years. Our results also reveal that strong volcanic eruptions like Eyjafjallajökull in 2010 have an important role in redistributing anthropogenic radionuclides from the stratosphere to the troposphere. Anthropogenic radionuclides have been injected into the atmosphere by nuclear weapon tests (NWT) in the fifties, sixties and seventies, the burn-up of the SNAP-9A satellite [1] , and accidents in nuclear power plants such as Chernobyl (1986) and Fukushima (2011). Radioactive debris became rapidly attached to ambient aerosol particles, which determined the mechanisms governing their atmospheric transport. In the troposphere, dry and wet deposition removes most contaminants within a few weeks to months. In the stratosphere, mean residence time for radioactive debris is longer due to the thermal stratification and separation from the troposphere by the tropopause and the smaller size distribution of the aerosols [2] . It is generally accepted that the current level of plutonium (Pu) in the stratosphere is negligible and that the tropospheric level is mainly controlled by resuspension of Pu-bearing particles deposited on land [3] , [4] , [5] , [6] , [7] , [8] , [9] . There are, however, limited available data on radionuclide transport and distribution in the stratosphere, the size distribution of the radioactive particles and its interaction with natural aerosols. Most information comes from early studies in the sixties and seventies on anthropogenic radionuclides in the atmosphere [10] , [11] , [12] , [13] , [14] , [15] , [16] , [17] , [18] . In these studies, tropospheric and stratospheric aerosols were sampled with the aid of aircraft and balloons. Because of the significant decrease in the atmospheric level of most radionuclides, as a consequence of the introduction of the Nuclear Test Ban Treaty (NTBT) in 1963, most laboratories abandoned stratospheric surveillance in the early eighties. The collected radionuclide data were nonetheless very useful for investigating atmospheric processes [19] . Results show that the transfer of radioactive debris from the stratosphere to the troposphere takes place mainly at the tropopause breaks, with a maximum in spring and a minimum in autumn [13] , [16] , [20] . Radioactive particles in the size range of 1–10 μm settle rapidly out of the stratosphere with mean residence times of the order of weeks to months [2] , [12] , [21] . However, the bulk of stratospheric radioactivity was associated with particles below a few tenths of a micrometre in radius (<0.1 μm) and persisted in the stratosphere for years [2] , [20] . Radioactive particles with radius below 0.02 μm were typically found above 27 km, and particles of larger radius were found between the tropopause and 21 km. Mean residence times of the order of 1–4 years were reported for radioactive particle aerosols in the stratosphere [2] , [13] , [15] , [16] , [20] . These estimations were based on the rates of change of the stratospheric burden over short timescales (2–4 years), and numerous important factors/parameters were not taken into account. We could mention, for example, transport processes in the stratosphere (for example, horizontal mixing, interhemispheric transfer), the longer residence times for small particles (older tail of a residence time distribution) and the effect of stratospheric mixing of debris from different NWTs. Other studies on Pu radionuclides and 137 Cs in the atmosphere are based mainly on monitoring their long-term evolution in surface aerosols and atmospheric depositions. These studies have consistently suggested that Pu activities in the stratospheric compartment may have decayed with mean residence times of 1.0–1.7 years [22] , [23] , [24] , [25] . The general mixing of stratospheric with tropospheric air is the main mechanism of NWT deposition. However, Pu activity in the stratosphere is not controlled by the same processes as in the troposphere. Several studies have shown that Pu in ground-level air is strongly influenced by resuspension of Pu in soil particles [6] , [7] , [26] , [27] , [28] , [29] . Hence, the estimation of a mean residence time of Pu in the stratosphere by this approach may have been biased to lower values. High-altitude aerosols (from 8 to 13 km above sea level) have been collected periodically since 1970 under the framework of the environmental radioactivity survey of Switzerland with the aid of aircraft [30] , [31] . Elevated concentrations of anthropogenic radionuclides were detected in tropospheric aerosol samples after the passage over Switzerland of the ash plume of the Eyjafjallajökull volcano eruption in 2010. Activities of Pu and 137 Cs were, for example, up to three orders of magnitude higher than the levels reported for ground-level aerosols [30] . These were surprising results and at first glance contradicted previous studies on radionuclides in the atmosphere. The purpose of this work is to measure Pu, 241 Am and 137 Cs in air filters from different layers of the troposphere (ground level to upper troposphere) and the lower level of the stratosphere with the aim to determine the residence time of both radionuclides in the atmosphere. We use a 241 Am/ 241 Pu age-dating model to determine the time of the introduction of Pu into the atmosphere. In addition, we study the effect of the volcanic eruption of the Eyjafjallajökull volcano of 2010 to reveal the potential role of volcanic eruptions on the redistribution of radioactive contamination present in the atmosphere. 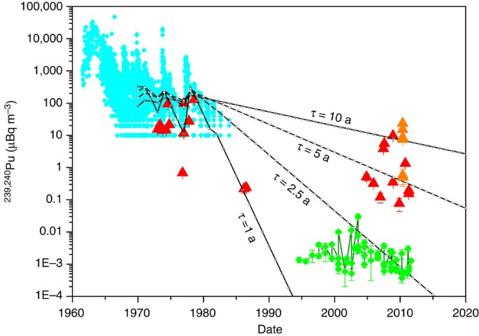Figure 1: Activity concentration of239,240Pu in the atmosphere. 239,240Pu in stratospheric aerosols from Switzerland (red traingles) and in aerosols samples from the high-altitude aerosol monitoring programmes of the Environmental Measurements Laboratory (light blue rhombus): stardust, airstream and ashcan11,14,17,18.239,240Pu in the Eyjafjallajökull volcano ash plume (orange triangles) and at ground-level air in Switzerland (green rhombus) are also shown. The lines represent the Pu distribution obtained by the exponential model for different mean residence times (τ=1, 2.5, 5 and 10 a). Uncertainties are expressed at 95% level of confidence (k=2). Anthropogenic radionuclides in the atmosphere The activities of 239,240 Pu in stratospheric and tropospheric aerosols over Switzerland are displayed in Table 1 . Graphical representation of 239,240 Pu and 137 Cs in stratospheric and tropospheric aerosols as a function of the year of collection over Switzerland are shown in Figs 1 and 2 . 239,240 Pu activities in stratospheric aerosols of Switzerland in the seventies were comparable to the activities reported by the Stardust, Airstream and Ashcan high-altitude sampling programmes of the Environmental Measurements Laboratory ( Fig. 1 ) [11] , [14] , [17] , [18] . 239,240 Pu and 137 Cs in the stratosphere have since steadily decreased, and current levels are down to two orders of magnitude lower than the ones measured in 1974 ( Fig. 1 ). 239,240 Pu activities in stratospheric aerosols are nonetheless up to five orders of magnitude higher than in ground-level aerosols at present days ( Fig. 1 ). 137 Cs behaved similarly, with high-altitude aerosols having up to three orders of magnitude higher activities than ground-level aerosols ( Fig. 2 ). Table 1 Activities of 239,240 Pu in high-altitude aerosol samples from Switzerland. Full size table Figure 1: Activity concentration of 239,240 Pu in the atmosphere. 239,240 Pu in stratospheric aerosols from Switzerland (red traingles) and in aerosols samples from the high-altitude aerosol monitoring programmes of the Environmental Measurements Laboratory (light blue rhombus): stardust, airstream and ashcan [11] , [14] , [17] , [18] . 239,240 Pu in the Eyjafjallajökull volcano ash plume (orange triangles) and at ground-level air in Switzerland (green rhombus) are also shown. The lines represent the Pu distribution obtained by the exponential model for different mean residence times ( τ =1, 2.5, 5 and 10 a). Uncertainties are expressed at 95% level of confidence ( k =2). 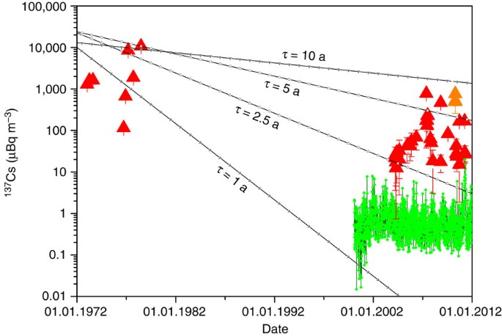Figure 2: Activity concentration of137Cs in the atmosphere. 137Cs in low tropospheric (green rhombus) and stratospheric (red triangles) aerosols of Switzerland.137Cs in the Eyjafjallajökull volcano ash plume is also shown (orange triangles). The lines represent the137Cs distribution obtained by the exponential model for different mean residence times (τ=1, 2.5, 5 and 10 a). Uncertainties are expressed at 95% level of confidence (k=2). Full size image Figure 2: Activity concentration of 137 Cs in the atmosphere. 137 Cs in low tropospheric (green rhombus) and stratospheric (red triangles) aerosols of Switzerland. 137 Cs in the Eyjafjallajökull volcano ash plume is also shown (orange triangles). The lines represent the 137 Cs distribution obtained by the exponential model for different mean residence times ( τ =1, 2.5, 5 and 10 a). Uncertainties are expressed at 95% level of confidence ( k =2). Full size image Activity and isotopic ratios of radionuclides We used the 241 Am/ 241 Pu age-dating method [32] on selected aerosol samples to corroborate the time of the introduction of Pu in the atmosphere. The calculated dates showed consistently that the Pu contamination occurred between 1964 and 1982 ( Table 2 ). Activity ratios, recalculated to the date of sampling, of 12–14 for 241 Pu/ 239,240 Pu and 240 Pu/ 239 Pu isotope ratios close to 0.18 ( Table 2 ) are also consistent with the ratios reported in atmospheric aerosols after the NTBT in 1963 (ref. 1 ). This is corroborated by 241 Am/ 239,240 Pu ratios close to 0.5. 238 Pu/ 239,240 Pu ratios higher than expected for NWT fallout (typical ratios of 0.02–0.03) suggest additional Pu sources ( Fig. 3 ). Enriched 238 Pu in the stratosphere was observed during the years after the burn-up of the 238 Pu-powered satellite SNAP-9A at about 50 km in the atmosphere in 1964 (ref. 15 ). This event increased significantly the amount of 238 Pu in the atmosphere ( Fig. 3 ). The relatively high 238 Pu/ 239,240 Pu activity ratios observed currently indicates that 238 Pu originating mainly from the satellite accident and from NWT with high 238 Pu/ 239,240 Pu, possibly injected in the upper stratosphere, is still circulating in the stratosphere. A 239,240 Pu/ 137 Cs mean activity ratio of 0.0118 was found in post-moratorium (NTBT) stratospheric aerosols ( Fig. 4 ), which is in good agreement with the average 239,240 Pu/ 137 Cs activity ratio of 0.012 reported for global fallout [33] , [34] . Nevertheless, recent 239,240 Pu/ 137 Cs activity ratios in stratospheric aerosols deviate significantly from the above correlation line ( Fig. 4 ). This may be explained by their different chemical/physical properties (for example, volatilities, particle affinities in the atmosphere and so on). Table 2 Activities of 241 Pu and 241 Pu/ 239,240 Pu activity ratios in high-altitude aerosol samples from Switzerland. 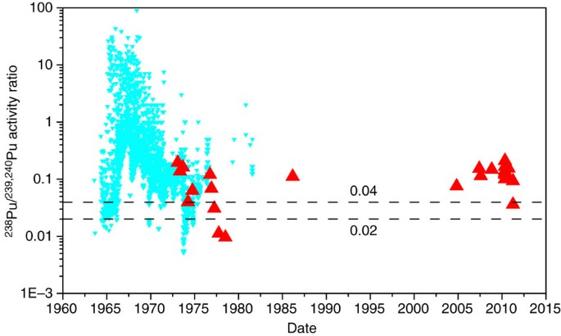Figure 3:238Pu/239,240Pu activity ratios in stratospheric aerosols. Activity ratios in stratospheric aerosols from Switzerland (red traingles) and in aerosol samples from the high-altitude aerosol monitoring programmes of the Environmental Measurements Laboratory (light blue triangles): stardust, airstream and ashcan11,14,17,18. The dashed lines at 0.02 and 0.04 represent the current range of238Pu/239,240Pu activity ratios in ground-level aerosols and soil samples from Switzerland. Full size table Figure 3: 238 Pu/ 239,240 Pu activity ratios in stratospheric aerosols. Activity ratios in stratospheric aerosols from Switzerland (red traingles) and in aerosol samples from the high-altitude aerosol monitoring programmes of the Environmental Measurements Laboratory (light blue triangles): stardust, airstream and ashcan [11] , [14] , [17] , [18] . The dashed lines at 0.02 and 0.04 represent the current range of 238 Pu/ 239,240 Pu activity ratios in ground-level aerosols and soil samples from Switzerland. 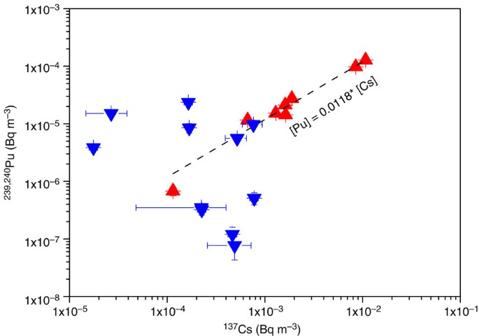Figure 4: Correlation between239,240Pu and137Cs in stratospheric aerosols. Red triangles represent the post-moratorium (after the NTBT in 1963) stratospheric aerosols (1973–1986). Blue triangles represent recent stratospheric samples taken after 2004.The correlation line for the post-moratorium samples is also shown. Full size image Figure 4: Correlation between 239,240 Pu and 137 Cs in stratospheric aerosols. Red triangles represent the post-moratorium (after the NTBT in 1963) stratospheric aerosols (1973–1986). Blue triangles represent recent stratospheric samples taken after 2004.The correlation line for the post-moratorium samples is also shown. Full size image The determination of radioelement isotopic ratios and the 241 Am/ 241 Pu-dating method all confirmed that Pu contamination in the stratosphere was mainly originated from the NWTs fallout and the burn-up of the satellite SNAP-9A. Over the past decades, stratospheric 239,240 Pu and 137 Cs activities showed a large variability that suggests a low mixing rate of stratospheric air masses and/or the input of these radionuclides from upper layers of the stratosphere. The lower variability observed in ground-level air may indicate that equilibrium or steady-state conditions have been reached for the sources (for example, resuspension, transfer from the stratosphere) and sinks (for example, deposition) of these radionuclides in the troposphere. Our results show that significant fractions of radioactive aerosols (possibly small particles <0.1 μm) remain in the stratosphere for timescales of the order of several decades. Mean residence time of stratospheric air can be obtained from observations of tracer changes in the atmosphere [35] , [36] , [37] , [38] , [39] , [40] , [41] . We used an exponential distribution model (box model) to interpret the trend of Pu and 137 Cs in the stratosphere of Switzerland. This choice was justified by the sparse data set of Pu and 137 Cs in stratospheric aerosols, which is not suitable for estimating annual trends. In addition, the distributions of our data sets fit well the asymmetric shape of the exponential distribution, with a peak for short residence times and a long tail for long residence times. The radionuclide is assumed to be distributed homogeneously over the stratospheric domain. The model does not resolve the spatial distribution of the radionuclide within the stratospheric domain, but it describes the activity of the radionuclide (for example, 239,240 Pu, 137 Cs) inside a box representing the stratosphere over Switzerland. We assumed that horizontal inflow and outflow of the radionuclide into the box are similar. However, vertical downward transport from upper layers of the atmosphere into the stratospheric box and out of the box through the tropopause may have strong effects on the radioisotope activity and therefore on the mean age of the tracer. Best agreement between the measured and modelled Pu activities were obtained for mean residence times of Pu in the stratosphere of 2.5–5 years ( Fig. 1 ). The mean residence times were further confirmed by the 137 Cs data ( Fig. 2 ). These results are in good agreement with previous estimations of the mean residence time of stratospheric air using sampling methods like aircrafts, high-altitude balloons and satellite observations [35] , [38] , [40] . Radioisotopes introduced in the atmosphere as a consequence of the nuclear bomb tests during the fifties and sixties are still useful tracers to study transport processes. The aerosol samples collected in the low tropopause (altitude: 1–3 km) during the Eyjafjallajökull event showed Pu activities and 238 Pu/ 239,240 Pu activity ratios similar to the ones observed in stratospheric aerosols ( Figs 1 and 3 , Table 1 ). This result indicates that the Pu detected in the volcano ash plume may have come from the stratosphere. The Eyjafjallajökull is a sub-glacial volcano covered by an ice cap of about 77 km 2 , which is about 250 m thick at the summit of 1,666 m above sea level. During the eruption of April 2010, thousands of tons of molten rock came into contact with ice creating a huge explosion throwing steam and particles high into the air. This explosive eruption introduced volcanic fine-grained ash and gases (for example, SO 2 ) up to the lowermost stratosphere [42] , [43] . In the atmosphere, sulphur-bearing gases such as SO 2 transformed into tiny sulphuric acid particles [2] , [44] . Aerosol size distributions within ash clouds showed a fine mode (0.1–0.6 μm) associated with sulphuric acid and/or sulphate, and a coarse mode (0.6–35 μm) associated with ash [45] . Numerous studies showed that the Eyjafjallajökull ash particles were strongly depolarizing [46] and that particles were electrically charged [47] , [48] . Harrison et al . [47] proposed radioactive decay as a potential source for this particle depolarization. Charging of aerosols has significant effects on their transport mechanisms like changes in the vertical deposition speeds and particle–particle agglomeration rates [49] . Charged particles have, for example, increased collision efficiencies and therefore large scavenging coefficients [50] . We hypothesize that the introduction of ash particles and gases into the stratosphere by the Eyjafjallajökull volcano is responsible for an increased scavenging of Pu and 137 Cs aerosols in the stratosphere and an increased transport into the troposphere by sedimentation. This hypothesis is further supported by the presence of cirrus-like formations over Europe after the volcano eruption. Volcanic ash particles favour ice nucleation (IN). Seifert et al . [51] showed the existence of very efficient IN during the Eyjafjallajökull volcanic event. Bingemer et al . [52] also observed a large increase of the IN concentration during this event, with IN surface densities of at least a factor two higher than that in other conditions (for example, air masses affected by mineral dust). Seifert et al . [51] demonstrated the presence of ash-assisted formation of cirrus-like clouds in the troposphere over Leipzig and Maisach during several days after the first observational period (14–17 April 2010). This was further confirmed by the detection of a volcanic ash-induced cirrus cloud at altitudes of 8–11 km over Jülich during the passage of the Eyjafjallajökull ash plumes [46] . The backward trajectory analysis confirmed that the cirrus cloud was originated from ash loadings of air masses near Iceland [46] . The air masses had relative humidities slightly above 100% in which the formation of ice crystals was very favourable. The ash layer then descended with the cirrus cloud. Trickl et al . [43] concluded that a branch of the ash plume was present in the tropopause over Garmisch-Partenkirchen on 19 April, and that some volcanic contribution in the lowermost stratosphere cannot be excluded. Backward trajectories revealed Iceland as the closest source region for the air masses of the troposphere and lowermost stratosphere [43] . Trickl et al . [43] suggested that the cirrus formation occurred between 14 and 16 April 2013 in the upper troposphere over Iceland where favourable conditions for aerosol growth existed (relative humidity exceeded 80% several times). Here we show that the strong volcanic eruption of the Eyjafjallajökull volcano has redistributed anthropogenic radionuclides in the lower atmosphere. Waugh [38] emphasized the need for more measurements of ‘age tracers’. We believed that NWT radionuclides could be a very good proxy for the study of atmospheric air mass transfer during the last 50 years. In this respect, Pu is the perfect candidate because it has a long physical half-life and a high distribution coefficient on mineral and organic particles, and do not react with atmospheric components under light irradiation. Sampling and laboratory methods High-altitude aerosols were collected six times a year with especially prepared military airplanes. This sampling programme started in the seventies but it was interrupted between the end of the eighties and 2004 (ref. 31 ). Air volumes between 200 and 3,000 m 3 were filtered through cellulose filters (555 × 526 mm 2 , type 0048, Whatman). The filters were immediately analysed by gamma spectrometry [31] , [53] . Ground-level aerosols (at 1 m above the soil surface) were collected with high volume samplers (500–800 m 3 h −1 ) at five different locations of Switzerland. The samples were analysed by gamma spectrometry on a weekly basis. Since 1994, the cumulative samples of 1 year for each sampling location (annual air volumes >200,000 m 3 ) was analysed for alpha emitters. After the eruption of the Eyjafjallajökull volcano in 2010, aerosol samples were collected during the passage over Switzerland of the ash plume at the altitude of 1–3 km (ref. 30 ). In this study, we selected several samples of high-altitude aerosol for analysing Pu and 241 Am. The air filters were ashed at 550 °C for 48 h before the radiochemical analysis. The radiochemical method combined high-pressure microwave digestion for the dissolution of the ashes with the highly selective extraction chromatographic resins Tetravalent (TEVA, the extractant is a quaternary ammonium salt) and N,N,N′,N′-tetra-n-octyldiglycolamide (DGA) (supplied by Triskem International, Bruz, France) to purify Pu and americium [54] . The alpha sources were prepared by electrodeposition on stainless steel discs. High-resolution alpha spectrometry was performed on an alpha spectrometer with passivated implanted planar silicon (PIPS) detectors (Alpha Analyst, Canberra Electronic, France). Selected Pu alpha sources were redissolved in concentrated HNO 3 and HCl as described in ref. 32 for determining either the activity of 241 Pu by liquid scintillation counting (Quantulus 1220, Wallac) or the concentration of 239 Pu and 240 Pu by sector-field inductively coupled plasma mass spectrometry equipped with a desolvation unit for the reduction of 238 U 1 H molecular interference isobaric to 239 Pu. The inductively coupled plasma mass spectrometry analysis was carried out on an Element 2 at the Federal Office of Public Health according to ref. 55 . Age distribution model We have chosen an exponential distribution model to interpret our radionuclide data in stratospheric air. The response function of the exponential model ( g ( t )) is represented by where T represents the mean residence time of the distribution and t is the time. The whole residence time distribution, also named age spectra [38] , is only characterized by T , which represents in our study case the mean residence time of the radionuclide in the stratosphere. The initial activity of the radionuclide in the stratospheric box is set for the year 1970, a few years after the entry into force of the NTBT. The input of the radionuclide into the stratospheric layer in the seventies is calculated from the activity values reported by the Environmental Measurements Laboratory [11] , [14] , [17] , [18] . After 1980, any additional input of 239,240 Pu is assumed to be negligible. How to cite this article: Corcho Alvarado, J.A. et al . Anthropogenic radionuclides in atmospheric air over Switzerland during the last few decades. Nat. Commun. 5:3030 doi: 10.1038/ncomms4030 (2014).